Leg-tracking and automated behavioural classification inDrosophila Much remains unknown about how the nervous system of an animal generates behaviour, and even less is known about the evolution of behaviour. How does evolution alter existing behaviours or invent novel ones? Progress in computational techniques and equipment will allow these broad, complex questions to be explored in great detail. Here we present a method for tracking each leg of a fruit fly behaving spontaneously upon a trackball, in real time. Legs were tracked with infrared-fluorescent dyes invisible to the fly, and compatible with two-photon microscopy and controlled visual stimuli. We developed machine-learning classifiers to identify instances of numerous behavioural features (for example, walking, turning and grooming), thus producing the highest-resolution ethological profiles for individual flies. A major goal of biology is to elucidate the mechanisms underlying behaviour and how they have evolved. Because of its vast genetic toolkit, Drosophila melanogaster is an ideal model system for understanding the underpinnings of behaviour. However, analysing behaviour is not trivial and therefore most studies rely on simple, robust behaviours such as phototaxis [1] and olfactory chemotaxis [2] . Classic paradigms, performed on groups of flies, quantify these behaviours efficiently, but coarsely. In contrast, methods to efficiently characterize the behaviour of individual flies at high levels of detail are rare. With recent advances in computer vision, a new generation of automated and sophisticated assays are being developed that allow for richer characterizations of behaviours, and consequently the genes, circuits and evolution underlying them. The first high-resolution analysis of Drosophila walking was a labour-intensive, frame-by-frame movie analysis [3] . Newer, sophisticated techniques can automatically annotate behaviour at the level of conspicuous behaviours of single flies. For example, the most sensitive methods to date can track individual animals and detect the behavioural motifs of walking, lunging and wing extension, but cannot resolve individual legs [4] , [5] . Given the tiny size of Drosophila , legs are exceptionally difficult to track, particularly when flies are imaged within a large arena. Visualizing the legs is vital for identifying behaviours such as grooming or for a deeper analysis of walking. Using a total internal reflection based optical method, Mendes et al . [6] were able to achieve high temporal and spatial resolution of a walking fly, including its legs, to explore gait parameters in great detail. The legs of large insects, like cockroaches, marked with paint on their joints, have been tracked with high-speed cameras, and detailed analyses of their locomotion have been performed [7] . However, the data acquisition requires human assistance. Unfortunately, both of these methods only capture several seconds of walking because they require that the insect walks within the narrow field of view of the high-speed camera [6] , [7] . Recently, recordings for ~1 min of a freely behaving cricket with many paint markers on its body have been made using manual camera tracking and automated offline video analysis [8] . In contrast to such arena assays, tethered Drosophila walking behaviour assays (for example, Buchner [9] , Seelig et al . [10] , Clark et al . [11] and Gaudry et al . [12] ) can capture long periods (several hours) of data, but to date have not included the tracking of individual legs. Here we present a method that overcomes these limitations. It is the first technique that tracks in real time the six individual legs and the fictive movement of a tethered fruit fly behaving either spontaneously or in response to controlled visual stimuli, for hours. We also developed a machine-learning classifier that automatically detects and categorizes distinct behavioural features (for example, walking, turning and grooming), rapidly providing the most detailed behavioural recordings of single flies yet achieved. Notably, this setup was designed for compatibility with either electrophysiology or optophysiological two-photon microscopy. This approach exploits the near-infrared fluorescence of two oxazine dyes to visualize leg position with conventional (and economical) optical components and detectors, in a compact arrangement suitable as the stage of custom multi-photon microscopes. Using this device, we have uncovered new insights about Drosophila behaviour. Specifically, we discovered significant individual-to-individual variation in freely behaving animals, and we found that individual variation is amplified by breaking the loop between motor behaviour and sensory feedback. Recording individual fly behaviour at high resolution We started with a traditional floating-ball treadmill rig [9] , [10] , [11] , [12] because tethering a behaving fly simplifies leg imaging and permits the future incorporation of simultaneous electrophysiology or optophysiology. We substituted a transparent ball to allow imaging of the legs from below using a custom imaging system ( Fig. 1a , Supplementary Fig. S1 ; Supplementary Methods ). The sphere was tracked by two infrared laser sensors normally found in computer mice. As each sensor only detects two dimensions of motion, two sensors were used to capture all three rotational components (pitch—the result of forward/backward running; yaw—the result of turning in place; and roll—the result of sidestepping/crabwalking) ( Supplementary Fig. S1d–f ; Supplementary Methods ). 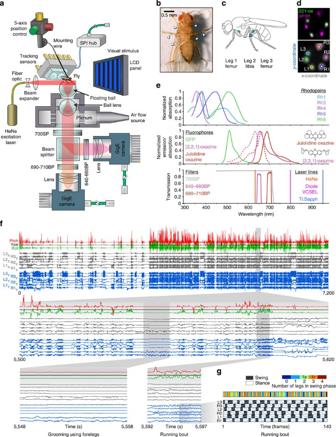Figure 1: The leg-tracker apparatus and its properties. (a) Schematic of the leg-tracker apparatus. A fly is mounted by wire tether to a clear sphere supported by flowing air. Fictive motion of the fly is recorded by tracking sensors. The dye spots on the leg fluoresce when excited by the HeNe laser and a second sphere re-collimates the image of the dye spots that are tracked from below by two cameras. (b) Photograph of a fly with bits of 221ox and julox dyes (arrowheads) glued alternately on each leg. (c) Cartoon illustrating the positioning of the dye spots. Dye was placed upon the femurs of the fore and hind limbs and upon the tibia of the middle legs. (d) Imaging of dye spots and detection of their positions. Top panel shows differential detection of alternating legs marked with the two dyes. Because the dyed segments on the front and hind legs do not cross, leg identity can be readily inferred in single frames (bottom panel). (e) Diagram of the absorption wavelengths of theDrosophilarhodopsins (top). Diagram of the absorption (dashed lines) and emission (solid lines) wavelengths of the 221ox and julox dyes and their chemical structures (middle). The dyes are compatible with green fluorescent protein (GFP). Emission wavelengths of the HeNe laser, vertical cavity surface emitting laser (VCSEL) of the tracking sensors and Ti:Sapphire lasers are depicted as vertical lines (bottom). Also shown are the transmission properties of the rig dichroic filters. (f) Representative data showing the 15 data vectors (3 for ball motion and 12 for leg positions) being recorded over 7,200 s (top). Magnification of a 120s data slice (middle). Higher magnifications of two typical behaviours (bottom). Red, black and green traces represent the ball’s pitch, yaw and roll components, respectively. Grey and blue traces are thexandycoordinates, respectively, of each leg. Plots are in arbitrary units, with ball motion vectors and leg-position components respectively comparable. Instrument output is calibrated. (g) Analysis of swing and stance phases during the second half of the running bout magnified inf. Blue lines correspond to the last six data vectors inf. Colour bar indicates the number of legs in swing phase at each frame, that is, the gait index—with Te indicating tetrapod gait (green) and Tr indicating tripod gait (orange). Figure 1: The leg-tracker apparatus and its properties. ( a ) Schematic of the leg-tracker apparatus. A fly is mounted by wire tether to a clear sphere supported by flowing air. Fictive motion of the fly is recorded by tracking sensors. The dye spots on the leg fluoresce when excited by the HeNe laser and a second sphere re-collimates the image of the dye spots that are tracked from below by two cameras. ( b ) Photograph of a fly with bits of 221ox and julox dyes (arrowheads) glued alternately on each leg. ( c ) Cartoon illustrating the positioning of the dye spots. Dye was placed upon the femurs of the fore and hind limbs and upon the tibia of the middle legs. ( d ) Imaging of dye spots and detection of their positions. Top panel shows differential detection of alternating legs marked with the two dyes. Because the dyed segments on the front and hind legs do not cross, leg identity can be readily inferred in single frames (bottom panel). ( e ) Diagram of the absorption wavelengths of the Drosophila rhodopsins (top). Diagram of the absorption (dashed lines) and emission (solid lines) wavelengths of the 221ox and julox dyes and their chemical structures (middle). The dyes are compatible with green fluorescent protein (GFP). Emission wavelengths of the HeNe laser, vertical cavity surface emitting laser (VCSEL) of the tracking sensors and Ti:Sapphire lasers are depicted as vertical lines (bottom). Also shown are the transmission properties of the rig dichroic filters. ( f ) Representative data showing the 15 data vectors (3 for ball motion and 12 for leg positions) being recorded over 7,200 s (top). Magnification of a 120s data slice (middle). Higher magnifications of two typical behaviours (bottom). Red, black and green traces represent the ball’s pitch, yaw and roll components, respectively. Grey and blue traces are the x and y coordinates, respectively, of each leg. Plots are in arbitrary units, with ball motion vectors and leg-position components respectively comparable. Instrument output is calibrated. ( g ) Analysis of swing and stance phases during the second half of the running bout magnified in f . Blue lines correspond to the last six data vectors in f . Colour bar indicates the number of legs in swing phase at each frame, that is, the gait index—with Te indicating tetrapod gait (green) and Tr indicating tripod gait (orange). Full size image Small pieces (~100 × 100 × 50 μm 3 ) of the dyes [2.2.1]-oxazine (221ox) [13] and julolidine-oxazine (julox) dye [14] were glued in alternation to each of the six legs ( Fig. 1b ; Supplementary Methods ). Flies were allowed to adapt to the dye spots for at least 24 h, and then mounted above the floating sphere via a wire tether glued to the thorax. A HeNe laser illuminated the dye on the legs, which were imaged from below, through the clear sphere, by two cameras ( Fig. 1a ). Each camera was equipped with a band-pass filter optimized for either 221ox or julox, allowing each leg to be uniquely detected, and adjacent legs distinguished ( Fig. 1d ). The optical wavelengths used here (between 630 and 850 nm) were chosen for their invisibility to the flies [15] —which exhibited no conspicuous responses to illumination—and compatibility with two-photon and traditional fluorescent microscopy ( Fig. 1e ). Animals were typically recorded in the dark for 2 h, although we have observed flies to behave beyond 16 h. After data acquisition, the fly can easily be removed from the tether and saved for future use. Custom LabView software records 15 vectors in real time: the x and y coordinates of each of the six legs, and the three rotational components of the floating sphere. The HeNe laser warmed the fly and ball slightly (increasing temperature 0.6 °C; see Supplementary Methods ). However, neither this temperature difference nor the presence of the dye spots had any discernible effect on behaviour, by eye, or as measured by the motion of the ball; (1) the distribution of pitch motion in the floating ball, (2) the intervals between bursts of pitch motion in the floating ball and (3) the auto-correlation properties of ball pitch motion, for flies that were unilluminated by the laser and unmarked with the dye, fell within the range seen for dyed and illuminated flies (and near their median; Fig. 2 ). 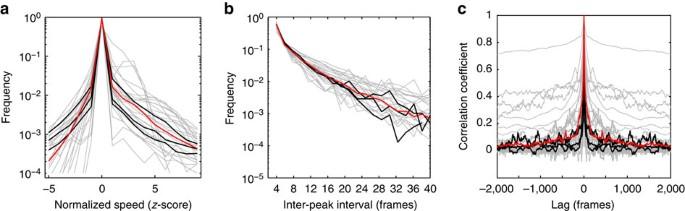Figure 2: Comparison of ball motion in dyed and undyed flies. (a) Histogram of normalized forward running speeds (ball pitch) from 2-h trials for normally dyed flies with the HeNe laser on (grey,n=27) and undyed flies with the HeNe laser off (black,n=3). Red indicates the median of dyed flies. (b) Histogram of intervals between peaks of forward running (ball pitch). Experiments and plot colouring as ina. (c) Auto-correlation plots for ball pitch vectors. Experiments and plot colouring as ina. Figure 2: Comparison of ball motion in dyed and undyed flies. ( a ) Histogram of normalized forward running speeds (ball pitch) from 2-h trials for normally dyed flies with the HeNe laser on (grey, n =27) and undyed flies with the HeNe laser off (black, n =3). Red indicates the median of dyed flies. ( b ) Histogram of intervals between peaks of forward running (ball pitch). Experiments and plot colouring as in a . ( c ) Auto-correlation plots for ball pitch vectors. Experiments and plot colouring as in a . Full size image Representative data is shown in Fig. 1f (see Supplementary Fig. S1g and Supplementary Methods ), including instances of grooming and running behaviours. From this data, we can reiterate previous gait analysis findings, such as identifying when the animal’s gait includes two or three legs simultaneously in swing phase (defined as tetrapod and tripod gaits, respectively). We find that fast running comprises primarily tripod gait [3] with brief excursions into tetrapod and non-canonical gaits [6] , the detection of which is largely a consequence of high temporal resolution ( Fig. 1g ). In addition to directly observing single leg strides via the dye and optics, the sphere itself was also responsive to single leg strides ( Supplementary Fig. S1h ). Automated classification of behaviour As our method records the position of legs at all times, we wanted to characterize behaviours other than running, such as grooming. Because of the volume of data collected (15 vectors per frame at 80+ Hz), we wanted to develop an automatic method for scoring behaviour. Non-linear classifiers have been quite successful at categorizing ethological data (see, for example, Dankert et al . [4] , Branson et al . [5] , Belongie et al . [16] , Veeraraghavan et al . [17] , Jhuang et al . [18] and Burgos-Artizzu et al . [19] ). After exploring support vector machines and neural network classifiers, we chose to pursue k -nearest neighbours (KNN) analysis ( Fig. 3a ; Supplementary Methods ) [20] , which had the advantage of conceptual simplicity and performance comparable to the other methods. Briefly, KNN works by placing an unclassified data point into a space with all the data points whose classifications are known (the training set). The classification applied to the plurality of the k neighbours (from the training set) nearest to the unclassified point is taken as the label of that point. To train the classifier, two investigators independently scored, frame-by-frame, movies recorded concurrently with leg tracking ( Fig. 3b ). The training set consisted of data from three male and two female flies; across these and all other animals examined, we observed no conspicuous sex-dependent behavioural differences. Training data needs to be generated only once and can be used to score all future trials. 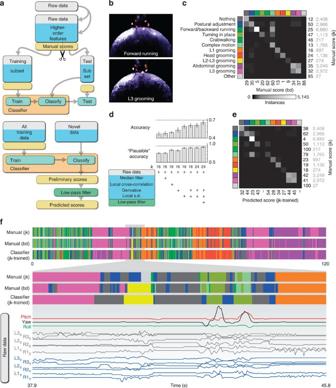Figure 3: KNN classifier for the automatic labelling of data. (a) Flowchart depicting development of the classifier (top) and its use to classify data (bottom) (see alsoSupplementary Methods). (b) Examples of movie frames used to hand-score behaviour for training the classifier. (c) Contingency matrix of the hand-scored movie-frame data sets from the two researchers. Shade of grey indicates the abundances of (dis)agreement between the two researchers. Colours here and ineandfindicate behaviour types. Black numbers at right and bottom, respectively, indicate the false-negative and false-positive rates (%) for each behavioural category with respect to the JK manual scoring. Grey numbers indicate the total number of frames manually annotated with each behaviour. (d) Including higher-order features with the raw data increases the classifier’s accuracy (accuracy was measured as the total fraction of frames scored correctly, that is, the unbalanced accuracy; seeSupplementary Methods). Behaviours such as forward/backward running and complex motion are qualitatively contiguous; the ‘plausible’ accuracy metric ignores errors between such pairs of behaviours (see text). Cross-validated error bars are ±s.e.m. calculated acrossn=5 flies. (e) Contingency matrix of the JK hand-scored data set to the classifier trained on the JK-scored data set. Numbers as inc. (f) Sequences of behaviour scores from both JK and BD manual data sets and from the classifier for the same 120-s window (top). Magnification of a ~8-sec subset along with the raw data used by the classifier (bottom). Figure 3: KNN classifier for the automatic labelling of data. ( a ) Flowchart depicting development of the classifier (top) and its use to classify data (bottom) (see also Supplementary Methods ). ( b ) Examples of movie frames used to hand-score behaviour for training the classifier. ( c ) Contingency matrix of the hand-scored movie-frame data sets from the two researchers. Shade of grey indicates the abundances of (dis)agreement between the two researchers. Colours here and in e and f indicate behaviour types. Black numbers at right and bottom, respectively, indicate the false-negative and false-positive rates (%) for each behavioural category with respect to the JK manual scoring. Grey numbers indicate the total number of frames manually annotated with each behaviour. ( d ) Including higher-order features with the raw data increases the classifier’s accuracy (accuracy was measured as the total fraction of frames scored correctly, that is, the unbalanced accuracy; see Supplementary Methods ). Behaviours such as forward/backward running and complex motion are qualitatively contiguous; the ‘plausible’ accuracy metric ignores errors between such pairs of behaviours (see text). Cross-validated error bars are ±s.e.m. calculated across n =5 flies. ( e ) Contingency matrix of the JK hand-scored data set to the classifier trained on the JK-scored data set. Numbers as in c . ( f ) Sequences of behaviour scores from both JK and BD manual data sets and from the classifier for the same 120-s window (top). Magnification of a ~8-sec subset along with the raw data used by the classifier (bottom). Full size image Hand scoring consisted of assigning to each frame of the movie one of the 12 possible behavioural labels ( Fig. 3c ). The definitions of these behavioural labels were not explicitly enumerated before scoring so that we could assess the degree of labelling discrepancies between investigators working independently—the appropriate benchmark for the automated training methods to follow. The two investigators achieved an unbalanced accuracy of 71%—that is, assigning the same score to 71% of frames, setting the goal for classifier performance ( Fig. 3c ). The greatest discrepancies between manual scorers appear between pairs of behaviours only distinguishable by arbitrary cutoffs (for example, complex motion versus forward/backward motion), as well as between abdominal and L3 grooming. The latter ambiguity reflects biological reality—we have observed flies to perform both of these behaviours simultaneously, stroking their abdomen as well as their hind legs. There was also a trend that rarer behaviours were scored less consistently between manual scorers. Classifiers trained on the original 15 vectors (the raw data) were mediocre (47% accuracy). However, augmenting the raw data with higher-order features, specifically the derivatives and local standard deviations of each of the 15 raw data vectors substantially improved performance (to 61% accuracy, see Supplementary Methods for calculations). Lastly, applying a low-pass filter to the classifier predictions further improved their accuracy. In the end, the classifier had an error rate only 5% greater than that seen between independent manual scoring (66% accuracy, Fig. 3d , see Supplementary Methods and Supplementary Movie 1 ). The accuracy was quite good (91%), if errors between behavioural categories that are only distinguishable by arbitrary cutoffs (the most common discrepancies in the manual scores) are ignored (see ‘plausible accuracy’ in Fig. 3d ). Fly-behavioural idiosyncrasy With the classifier in hand, we categorized the behaviour of individual flies (for example, Supplementary Movie 2 ) across 2-h trials. Flies spent most of their time pausing or grooming and ran more at the start of trials ( Fig. 4a ). We built ethograms [21] to look at the direction and frequency of transitions between the 12 behavioural types ( Supplementary Methods ). We found that the most frequent transitions were between the two types of foreleg grooming and the two types of hind-leg grooming ( Fig. 4d ). As has been reported in higher-level insect behaviours—for example, escape response [22] or phototaxis [23] , individual flies also showed variation in their behaviours. For example, one animal transitioned frequently from abdomen grooming to hind-leg grooming, whereas another animal did so more rarely. In contrast, the latter animal frequently alternated between abdomen grooming and pausing, whereas the former did so rarely ( Fig. 4d ). 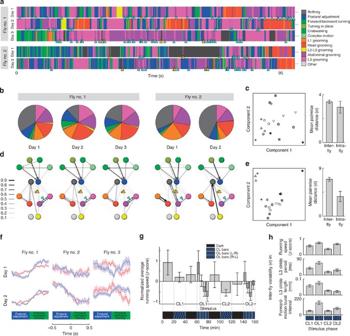Figure 4: The behavioural patterns of individual animals. (a) Multi-colour bars show snapshots (95 s) of classifier scores for multiple trials of two individual flies. Blue triangles indicate a behavioural transition more frequent in fly no. 1 and yellow triangles indicate a transition more frequent in fly no. 2. Colours here and inbanddindicate behaviour type. Ina–f, distinct trials for each fly were recorded on separate days. (b) Pie charts depicting fraction of time spent performing each behaviour for distinct trials from two individual animals, based on 2-h recordings per experiment per animal. (c) Left: spatial visualization of principal components (PCs) 1 and 2 underlying the inter-trial variance in fraction of time spent per behaviour inb. Shapes indicate multiple trials of an individual fly. Right: mean pairwise distance between and within flies in PC1–PC2 space at left. Bars are ±s.e.m. acrossn=153 inter-fly andn=12 intra-fly pairwise distances. SeeSupplementary Methods. (d) Ethograms of the same trials fromb. Arrows indicate direction of transition and thickness indicates frequency. Self-transitions are omitted for clarity. Triangles as ina. SeeSupplementary Methods. (e) Left: spatial visualization of principal components 1 and 2 underlying the variance in the ethograms fromd. Shapes indicate multiple trials across days of an individual fly. Right: mean pairwise distance between and within flies in PC1–PC2 space at left. Bars are ±s.e.m. acrossn=153 inter-fly andn=12 intra-fly pairwise distances. SeeSupplementary Methods. (f) Individuality in the averageycoordinates of the left (red) and right (blue) hind legs during the transition from postural adjustment to motion. Shaded regions indicate ±s.e.m., withnvarying according to the number of times each fly performed a postural adjustment–forward/backward running transition in each trial (48≤n≤282). (g) Running speed (z-score normalized across all experimental phases) during optomotor experiments as a function of stimulus. Bars are ±s.d. acrossn=5 flies. Blue/black patterns are representative top-to-bottom kymographs of the presented visual stimulus. CL, closed loop; OL, open loop. SeeSupplementary Methods. (h) Inter-fly variability (s.d.) of four different locomotor parameters, as a function of optomotor stimulus loop-closure status. Bar means in top graph correspond to error bars ing. The s.e. bars on the estimates of variability were determined by bootstrap resampling. L3 stride period and length were determined by inter-peak frequency analysis and are representative of all other legs. Forward-motion burst intervals were determined by the mode of the intervals between peaks of ball forward/backward velocity. Figure 4: The behavioural patterns of individual animals. ( a ) Multi-colour bars show snapshots (95 s) of classifier scores for multiple trials of two individual flies. Blue triangles indicate a behavioural transition more frequent in fly no. 1 and yellow triangles indicate a transition more frequent in fly no. 2. Colours here and in b and d indicate behaviour type. In a – f , distinct trials for each fly were recorded on separate days. ( b ) Pie charts depicting fraction of time spent performing each behaviour for distinct trials from two individual animals, based on 2-h recordings per experiment per animal. ( c ) Left: spatial visualization of principal components (PCs) 1 and 2 underlying the inter-trial variance in fraction of time spent per behaviour in b . Shapes indicate multiple trials of an individual fly. Right: mean pairwise distance between and within flies in PC1–PC2 space at left. Bars are ±s.e.m. across n =153 inter-fly and n =12 intra-fly pairwise distances. See Supplementary Methods . ( d ) Ethograms of the same trials from b . Arrows indicate direction of transition and thickness indicates frequency. Self-transitions are omitted for clarity. Triangles as in a . See Supplementary Methods . ( e ) Left: spatial visualization of principal components 1 and 2 underlying the variance in the ethograms from d . Shapes indicate multiple trials across days of an individual fly. Right: mean pairwise distance between and within flies in PC1–PC2 space at left. Bars are ±s.e.m. across n =153 inter-fly and n =12 intra-fly pairwise distances. See Supplementary Methods . ( f ) Individuality in the average y coordinates of the left (red) and right (blue) hind legs during the transition from postural adjustment to motion. Shaded regions indicate ±s.e.m., with n varying according to the number of times each fly performed a postural adjustment–forward/backward running transition in each trial (48≤ n ≤282). ( g ) Running speed ( z -score normalized across all experimental phases) during optomotor experiments as a function of stimulus. Bars are ±s.d. across n =5 flies. Blue/black patterns are representative top-to-bottom kymographs of the presented visual stimulus. CL, closed loop; OL, open loop. See Supplementary Methods . ( h ) Inter-fly variability (s.d.) of four different locomotor parameters, as a function of optomotor stimulus loop-closure status. Bar means in top graph correspond to error bars in g . The s.e. bars on the estimates of variability were determined by bootstrap resampling. L3 stride period and length were determined by inter-peak frequency analysis and are representative of all other legs. Forward-motion burst intervals were determined by the mode of the intervals between peaks of ball forward/backward velocity. Full size image This individual-to-individual variation could be an artifact of mounting bias. To examine this, we remounted the same individual flies on subsequent days. We found that the transition rates in the ethograms were significantly ( P =0.0022 and 0.0011 as estimated by t -test and bootstrap resampling, respectively; see Supplementary Methods ) more similar between re-mountings of the same fly than between flies, suggesting that much of the inter-trial variability comes from idiosyncrasies of the flies that persist for at least a few days ( Fig. 4e ). This was not observed (with statistical significance) in the simple percentage of time spent doing each behaviour ( Fig. 4c ), suggesting that there is more idiosyncrasy in the pairwise behavioural transition rates than in the overall off-rate of each behaviour. Moreover, the idiosyncratic nature of behavioural transitions is evident in fine-scale analysis of the mean positions of individual legs across said transitions ( Fig. 4f ). Thus, we conclude that certain ethological characterizations, namely the transitions between behaviours, are robust to any mounting artifacts, persist for days and vary across flies. As the setup uses wavelengths invisible to the fly ( Fig. 1e ), we can present controlled visual stimuli to the animal to study behaviours such as phototaxis or optomotor responses [24] . As a demonstration, we recorded animals’ responses to optic flow by placing them in front of a liquid–crystal display monitor displaying vertical bars translating from a line of expansion under either open- or closed-loop feedback control. We found that flies showed less variance in their average running speed during closed-loop trials relative to open-loop trials ( P =0.002, χ 2 -test of variance; Fig. 4g ), an effect also seen in measures of flight symmetry in ‘flight-simulator’ assays (Michael Reiser, personal communication). This pattern was also present in the inter-fly variability in leg-stride period, the intervals between bursts of pitch motion in the floating ball, and to a lesser extent stride length ( Fig. 3h ). We also observed that inter-fly variability generally diminished as the experiment proceeded. This method provides unprecedented level of detail for the characterization of walking behaviour, revealing rich and diverse behavioural profiles of individual animals. Using two dyes, two cameras and some optics, we were able to track each leg of a spontaneously behaving fruit fly in real time. With this technique, we observed that individual flies from the lab wild-type strain behaved idiosyncratically. The behavioural personality of an individual fly was consistent from day-to-day, at least over the time frame we examined. We also found that under closed-loop conditions, the flies behave more similarly to each other; perhaps interactive stimuli engage circuitry that overrides their more idiosyncratic preferences. The automatic classification of behaviour described here represents a general approach to developing automatic ethological classifiers for the efficient collection of statistically powerful data sets. This method will be a powerful tool for descriptive and comparative studies, for analysing subtle mutant phenotypes, and will reach its greatest potential upon integration with optophysiological recording, i.e. for probing the activity of neural circuits as they mediate individual behaviours. For example, the GAL4-targeted expression [25] of genetically encoded fluorescent physiological indicators [26] to neural subpopulations in the motor circuitry of the brain and ventral nerve cord, in simultaneous combination with leg and motion tracking, will be an effective technique for the identification of central pattern generators and decision-making circuitry. Fly stocks Flies (wild-type Canton S) were grown on standard cornmeal media (BuzzGro from Scientiis) in 25 °C incubators with a 12/12 h light–dark cycle. Behavioural experiments were recorded in an environmental room set at 23 °C, 40% humidity, with the lights off. Apparatus design details and use For the trackball, we used clear acrylic spheres (1/4′′; McMaster-Carr) suspended on air. The spheres were scuffed with sandpaper for better tracking by the infrared sensors. The two infrared sensors (Avago chip no. ADNS-6090) were extracted from high-performance gaming mice. See Supplementary Methods for additional design details. The x and y coordinates acquired from the two sensors were transformed to generate the three motion vectors of the sphere using trigonometry. See Supplementary Methods for details. For mounting, a fly was glued on the notum to a stainless steel no. 0 insect pin (Bioquip) using ultraviolet-cured adhesive (LED100 system from Electro-Lite Corporation and KOA 300 adhesive from Kemxert Corporation). The pin was glued to a flexible copper wire attached to a male audio jack. The male audio jack-wire-pin module was designed to be small and mobile so that it can be used at the dissecting scope. Once the fly was attached, the module press fits into a female audio jack that was attached to the micromanipulators (Siskiyou Inc) of the larger apparatus, which were used for fine adjustments to the animal’s position upon the sphere. Animals were allowed to adapt to their positioning in the device for approximately 20–40 min, in the dark, before data collection. The leg dyes were excited by a HeNe laser (632.8 nm; Thorlabs). The fluorescent light from the leg dye must pass through the clear trackball sphere to reach the imaging cameras (Prosilica GigE cameras; Allied Vision Technologies). Because this sphere will act as a lens, a second sphere is used to re-collimate the light before it reaches the cameras. Images were typically acquired at 80 Hz. Each camera used a band-pass filter (Edmund Optics) to optimize for the detection of one of the two leg dyes. In addition, a short-pass filter (NT49-829; Edmund Optics) was used to block stray light from the infrared tracking sensors and potential two-photon sources. See Supplementary Methods for additional details. Laser illumination warmed the fly and sphere slightly (0.6 °C), an effect less than that of the GigE cameras, which warmed the stage by 3 °C. Temperature effects were measured using a digital thermometer with a metal probe placed across the floating-ball socket, before and after 60 min of laser illumination. In real-time computational image processing, the 221ox image was masked out from the julox image within custom LabVIEW interfaces (National Instruments), so that the image from each camera now represented one specific tripod (that is, a set of three alternating legs). Leg identity was assigned by simple positional logic, for example, for the tripod consisting of the front-left, middle-right and back-left legs, the right-most image dot was assigned the identity of a middle leg, and the front-most of the remaining two dots a front-leg identity. We used a digital microscope video recorder (ProScope; Bodelin Technologies) for trials where movies were being simultaneously recorded for hand scoring. We inserted a polyester film filter (Roscolux, medium-blue colour filter no. 83; Roscoe Laboratories) over the microscope to block light from the HeNe laser while still allowing visualization of the sphere, fly and fluorescent dye spots. For the optomotor feedback experiments, we used a 15-inch liquid–crystal display monitor positioned 6 inches from the fly to display alternating blue- and black-coloured vertical bars. The trials comprised the conditions: 20 min in the dark; 20 min closed loop; 20 min dark; 20 min open loop; and repeat from the beginning once. Closed loop allowed the turns of the fly to control the position of the line of expansion for the translating vertical bars. See Supplementary Methods for additional details. Dyeing the fly legs The dye 221ox (phenoxazin-5-ium, 3,7-bis(7-azabicyclo[2.2.1]hept-7-yl)-chloride) was prepared according to the method described elsewhere [13] . The dye julox (1H,5H,11H,15H-diquinolizino[1,9-bc:1',9'-hi]phenoxazin-4-ium,2,3,6,7,12,13,16,17-octahydro-, chloride) was prepared according to the method described elsewhere [14] . Leg tracking would likely work using quantum dots [27] instead of the dyes, by selecting dots based on their diameters to match the emission spectra of the dyes, but we did not try this approach. The dyes were dissolved in methyl chloride and then mixed with clear nail polish and spread out into a thin film upon a glass slide to dry. Small pieces were cut out of the dye film with a scalpel. A small dab of ultraviolet-cured glue was placed on each leg of the animal under CO 2 anesthetization ( Fig. 1b ). A piece of dye film was placed onto the glue drop and then exposed to several seconds of ultraviolet light, thus securing the dye to the leg. Dye pieces were placed on the femurs of the fore and hind legs and the tibias of the middle legs to better separate the dye signals in space for easier tracking. Marked flies were allowed to recover and acclimate overnight. Raw data and analysis scripts All data from this project, as well as all LabView and MATLAB scripts, can be downloaded at: http://lab.debivort.org/leg-tracking-and-automated-behavioral-classification-in-Drosophila/. KNN classifier After exploring several types of classifiers, we settled on the KNN approach. Two researchers, independently, designated each frame of a movie as falling into one of the 12 behavioural types. Five movies (representing five distinct flies) comprising either 4,000 or 8,000 frames were scored. These behavioural annotations, in combination with the corresponding 15 raw data vectors, were used to train the classifier. Supplying higher-order features (such as the instantaneous leg motion velocities, for example) in addition to the raw data improved the classifier performance. See Supplementary Methods for more details on the development of the classifier. Data analysis Ethograms were calculated by populating a 12 × 12 transition matrix at position M a,b with the number of instances for which a frame of behaviour a precedes a frame of behaviour b . Self-transitions were ignored to focus on inter-behavioural transitions, and because the pie chart representations predominantly reflect self-transitions. Rows of the transition matrix were normalized by their totals to yield transition probabilities, which were visualized in a network fashion. Principle component analysis was performed on the (12) percentages of the pie charts and (132=12 × 11) probabilities of the ethograms, with replicates consisting of the 11 experiments done across five different flies over 2 days (or 3 days in the case of two flies). In both cases, all input variables were z -score normalized before principle component analysis, and the first two principle components were found to explain a minority of the total variance. Statistical significance of the clustering of each fly’s day-to-day replicates versus the overall distribution of the trials in Fig. 4c was determined in two ways: by t -test comparing the mean intra-fly distance in principal component (PC) space to the mean inter-fly distance; by a resampling approach in which the fly identity labels on the trial data were shuffled randomly and the intra-fly distances were re-calculated. The fraction of 50,000 trials in which the re-sampled mean intra-fly distance is less than or equal to the observed intra-fly distance is the P -value for this method, and was found to be in very close agreement with the t -test results. The intra-fly trials were not significantly clustered when total percentage of time in each behaviour was considered ( P =0.39 and 0.11 by t -test and resampling, respectively; Fig. 4c ), but were clustered when the transition rates between behaviours were considered ( P =0.0022 and 0.0011 by t -test and resampling, respectively; Fig. 4e ). The average position of each leg ( Fig. 4f ) was determined across behavioural transitions by identifying target behavioural transitions from the sequence of KNN-classified behaviours, and then averaging leg positions in a ±50 frame window flanking the transitions, across all occurrences of the transition. How to cite this article: Kain, J. et al . Leg-tracking and automated behavioural classification in Drosophila . Nat. Commun. 4:1910 doi: 10.1038/ncomms2908 (2013).